Photon energy upconversion through thermal radiation with the power efficiency reaching 16% The efficiency of many solar energy conversion technologies is limited by their poor response to low-energy solar photons. One way for overcoming this limitation is to develop materials and methods that can efficiently convert low-energy photons into high-energy ones. Here we show that thermal radiation is an attractive route for photon energy upconversion, with efficiencies higher than those of state-of-the-art energy transfer upconversion under continuous wave laser excitation. A maximal power upconversion efficiency of 16% is achieved on Yb 3+ -doped ZrO 2 . By examining various oxide samples doped with lanthanide or transition metal ions, we draw guidelines that materials with high melting points, low thermal conductivities and strong absorption to infrared light deliver high upconversion efficiencies. The feasibility of our upconversion approach is further demonstrated under concentrated sunlight excitation and continuous wave 976-nm laser excitation, where the upconverted white light is absorbed by Si solar cells to generate electricity and drive optical and electrical devices. The sun delivers light energy with 49% being in the infrared region [1] . A large fraction of infrared solar photons cannot be absorbed by photovoltaic cells working in the visible and near-infrared regions, such as commercially widely available Si-based and currently intensively researched perovskite solar cell [2] , [3] , as well as, by photocatalysts [4] and photoelectrocatalysts [5] active in the visible and near-infrared regions. This is because each infrared photon is too low in energy to promote desired electronic transitions in the semiconductors or molecules of the respective processes. Consequently, photon energy upconversion has been thought to be a promising way to the utilization of this portion of sunlight, by transforming two or more low-energy photons into a high-energy ones [2] , [6] , [7] . Photon energy upconversion from the infrared to visible region was first demonstrated in the early 1960’s by second-harmonic generation [8] and two-photon photoluminescence [9] , which require intense coherent excitation sources and deliver low-power conversion efficiencies. Coupled 4 f ions, benefiting from their ladder-like energy levels that facilitate photon absorption and subsequent energy transfer processes, offer higher power conversion efficiencies under moderate excitation densities through excited-state absorption or energy transfer upconversion [2] , [10] , [11] , [12] . Very recently, introduction of molecular dye sensitizers enables upconversion upon excitation within a broad absorption range of the dyes [13] . However, to the best of our knowledge, under continuous wave excitation, the highest power upconversion efficiency, defined as the output power of higher-energy photons divided by the input power of stimulating photons, is 12.7% (8.3% quantum yield) [14] . Intensive efforts are currently being made to synthesize upconversion materials with increasing power upconversion efficiencies [2] , [7] , [14] , [15] , [16] , [17] , [18] , [19] . In addition, there have been two recent studies with pulsed laser sources employed for excitation [20] , [21] , where the excitation power densities in each pulse are much higher than the corresponding time-averaged excitation power densities. The reported upconversion quantum yields are 16.2 and 16% and the corresponding power upconversion efficiencies are ~25 and 19%. A major factor limiting the efficiencies of energy transfer upconversion materials is multiphonon relaxation [22] , [23] , through which the excited electron energy dissipates to the crystal lattice as heat [17] . A process that can bypass or even benefit from multiphonon relaxation can potentially break the upconversion efficiency limit and hit higher efficiencies. Here, we demonstrate photon energy upconversion by thermal radiation. Ionic sensitizers are introduced to a host to absorb infrared photons and transfer energy to the host lattice through multiphonon relaxation [11] . Phonon accumulation in the host lattice boosts the temperature and intensifies the thermal radiation, for which a large fraction of photons have higher energy than the incident ones. This approach benefits from, rather than hindered by, multiphonon relaxation and therefore can reach very high efficiencies. The concept is verified with a variety of lanthanide and transition metal ion sensitizers and a variety of oxide hosts, from which guidelines are developed for designing materials with better upconversion performances. A power upconversion efficiency of 16% is achieved under continuous wave infrared excitation with 28 mol% Yb 3+ -sensitized ZrO 2 . The upconversion of low-energy solar photons into high-energy ones through thermal radiation is also demonstrated under direct concentrated sunlight excitation. Moreover, the upconverted white light under continuous wave laser excitation is illustratively transformed into electrical power with Si solar cells to drive optical and electrical devices. Upconversion with Yb 3+ -sensitized ZrO 2 We first examined the concept of photon energy upconversion ( Fig. 1 ) by thermal radiation with Yb 3+ -sensitized ZrO 2 . Yb 3+ is a typical near-infrared sensitizer owing to its absorption from 4 f electron 2 F 7/2 to 2 F 5/2 transition [24] . We chose ZrO 2 as the host for its high physical and chemical stability and optical transparency in the visible and near-infrared regions [25] . The highest phonon energy of ZrO 2 at 750 cm −1 enables the energy dissipation from excited-state electrons to the host lattice through multiphonon relaxation [11] , [26] . We prepared Yb 3+ -doped ZrO 2 using a sol–gel method. White powder ( Fig. 2a ) with irregular particle shapes ( Fig. 2c ) and an average particle size of 150±60 μm ( Supplementary Fig. 1 ) was obtained. For the doped ZrO 2 sample calcined at 800 °C, X-ray powder diffraction patterns ( Fig. 2e and Supplementary Fig. 2 ) can be indexed to the cubic phase [27] (JCPDS #: 81–1551) of ZrO 2 , when Yb 3+ concentration is between 8 and 40 mol% relative to the total molar amount of Yb and Zr. At low Yb 3+ concentrations from 1 to 5 mol%, the tetragonal phase (JCPDS #: 81–1545) dominates. Yb 3+ ions are uniformly distributed in the crystalline particle, as revealed by energy-dispersive X-ray elemental mapping ( Supplementary Fig. 3 ) on a scanning transmission electron microscope. 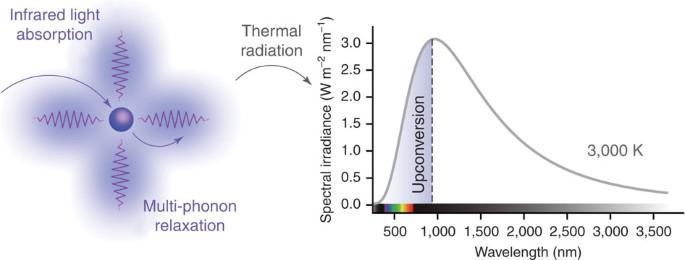Figure 1: Schematic showing photon energy upconversion by thermal radiation. Ionic sensitizers introduced to a host absorb infrared photons and transfer energy to the host lattice through multiphonon relaxation. Phonon accumulation in the host lattice causes thermal radiation. A large fraction of the emitted photons have higher energies than the incident ones. Figure 1: Schematic showing photon energy upconversion by thermal radiation. Ionic sensitizers introduced to a host absorb infrared photons and transfer energy to the host lattice through multiphonon relaxation. Phonon accumulation in the host lattice causes thermal radiation. A large fraction of the emitted photons have higher energies than the incident ones. 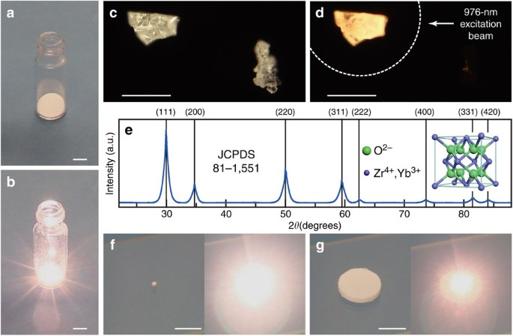Figure 2: Upconversion emission from 28 mol% Yb3+-doped ZrO2. (a) Photograph showing the sample to be white powder (scale bar, 5 mm). (b) Photograph of the powder sample excited by a collimated 976-nm laser beam (1.6 W, 760 W cm−2; scale bar, 5 mm). The sample glows. (c) Optical image of two irregularly shaped particles from the powder sample (scale bar, 200 μm). (d) Optical image of the same region, showing that one particle within the 976-nm laser beam (1.2 W, 570 W cm−2; scale bar, 200 μm) glows and the other particle outside the laser beam remains dark. (e) X-ray diffraction pattern of the sample calcined at 800 °C. The pattern can be indexed to the cubic phase (JCPDS #: 81–1551) of ZrO2. (f) Photographs of a sphere of 0.8 mm in diameter that glows under the 976-nm laser excitation (1.6 W, 760 W cm−2; scale bar, 5 mm). The sphere was fabricated by melting the powder sample in an arc melting furnace. (g) Photographs of a disk-shaped pellet of 8 mm in diameter that glows under the laser excitation at the same power (scale bar, 5 mm). The pellet was fabricated from the powder sample by mechanical pressing. Full size image Figure 2: Upconversion emission from 28 mol% Yb 3+ -doped ZrO 2 . ( a ) Photograph showing the sample to be white powder (scale bar, 5 mm). ( b ) Photograph of the powder sample excited by a collimated 976-nm laser beam (1.6 W, 760 W cm −2 ; scale bar, 5 mm). The sample glows. ( c ) Optical image of two irregularly shaped particles from the powder sample (scale bar, 200 μm). ( d ) Optical image of the same region, showing that one particle within the 976-nm laser beam (1.2 W, 570 W cm −2 ; scale bar, 200 μm) glows and the other particle outside the laser beam remains dark. ( e ) X-ray diffraction pattern of the sample calcined at 800 °C. The pattern can be indexed to the cubic phase (JCPDS #: 81–1551) of ZrO 2 . ( f ) Photographs of a sphere of 0.8 mm in diameter that glows under the 976-nm laser excitation (1.6 W, 760 W cm −2 ; scale bar, 5 mm). The sphere was fabricated by melting the powder sample in an arc melting furnace. ( g ) Photographs of a disk-shaped pellet of 8 mm in diameter that glows under the laser excitation at the same power (scale bar, 5 mm). The pellet was fabricated from the powder sample by mechanical pressing. Full size image On excitation with a collimated 976-nm laser beam at a spot size of 0.0021±0.0003, cm 2 , the powder sample emits bright white light to naked eyes ( Fig. 2b and Supplementary Movie 1 ), indicating visible photon emission under infrared photon excitation. Optical microscopy reveals that the individual particles glow within the excitation laser beam and function as emission centres ( Fig. 2d ; Supplementary Fig. 4 ; Supplementary Movies 2 and 3 ). Moreover, the powder sample can be fabricated into spheres ( Fig. 2f and Supplementary Fig. 5 ), pellets ( Fig. 2g ) and potentially arbitrary shapes by arc melting or pressing. After reshaping, the sample retains its upconversion capability ( Supplementary Fig. 5 and Supplementary Movie 4 ). Power upconversion efficiency To verify the thermal radiation nature of the light emission, we recorded the irradiance spectrum ( Fig. 3a ) from 300 to 1600, nm using two charge-coupled device cameras that were responsive in different spectral regions and coupled to the same spectrometer. Despite the different signal-to-noise ratios of the spectra taken with the different cameras, the entire spectrum can be well fitted to Planck’s law [28] with a blackbody temperature of 2,850 K ( Fig. 3a ). Increasing the excitation power density does not invalidate the Planckian radiation character but increases the blackbody temperature ( Fig. 3b,c ). 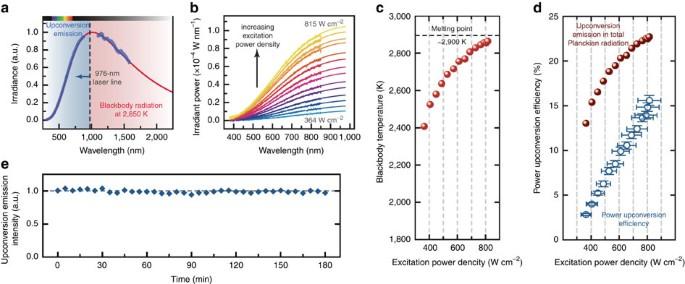Figure 3: Upconversion characteristics of 28 mol% Yb3+-doped ZrO2. (a) Irradiance spectrum (blue) of the sample under 976-nm excitation (1.7 W, 800 W cm−2). The irradiance spectrum fits well to Planckian radiation at 2,850 K (red). The blue-shaded area indicates the portion of the upconversion emission. (b) Irradiant powers recorded as the excitation power density was gradually increased from 364 to 815 W cm−2. Each spectrum was fitted according to Planck’s law to obtain the blackbody temperature. (c) Variation of the blackbody temperature with the excitation power density. The blackbody temperature increases monotonically, approaching the melting point of ZrO2. (d) Measured (open circles) and estimated (solid spheres) power upconversion efficiencies. The measured efficiency increases to 16% as the excitation power density reaches 800 W cm−2. The estimated efficiency refers to the percentage of the emission power at the higher-energy side of the excitation laser line in the total Planckian radiation power at a certain blackbody temperature. The full heights of the vertical and horizontal error bars correspond to one s.d. of the measured upconversion emission power and the excitation power density, respectively. The horizontal error bars arise mainly from the uncertainty of the laser spot size on the sample. (e) Upconversion emission intensity measured as a function of time, showing nearly no decay within 180 min under the continuous excitation of the 976-nm laser (1.6 W, 760 W cm−2). Figure 3: Upconversion characteristics of 28 mol% Yb 3+ -doped ZrO 2 . ( a ) Irradiance spectrum (blue) of the sample under 976-nm excitation (1.7 W, 800 W cm −2 ). The irradiance spectrum fits well to Planckian radiation at 2,850 K (red). The blue-shaded area indicates the portion of the upconversion emission. ( b ) Irradiant powers recorded as the excitation power density was gradually increased from 364 to 815 W cm −2 . Each spectrum was fitted according to Planck’s law to obtain the blackbody temperature. ( c ) Variation of the blackbody temperature with the excitation power density. The blackbody temperature increases monotonically, approaching the melting point of ZrO 2 . ( d ) Measured (open circles) and estimated (solid spheres) power upconversion efficiencies. The measured efficiency increases to 16% as the excitation power density reaches 800 W cm −2 . The estimated efficiency refers to the percentage of the emission power at the higher-energy side of the excitation laser line in the total Planckian radiation power at a certain blackbody temperature. The full heights of the vertical and horizontal error bars correspond to one s.d. of the measured upconversion emission power and the excitation power density, respectively. The horizontal error bars arise mainly from the uncertainty of the laser spot size on the sample. ( e ) Upconversion emission intensity measured as a function of time, showing nearly no decay within 180 min under the continuous excitation of the 976-nm laser (1.6 W, 760 W cm −2 ). Full size image The broad Planckian radiation band covers the entire visible and near-infrared region, with a significant portion located at the higher-energy side of the excitation laser line (blue shaded area in Fig. 3a ), suggesting a considerable ratio of the upconversion emission within the total Planckian radiation. This intrigued us to quantify the power upconversion efficiency, where an integrating sphere was utilized to collect all the diffuse emission from the powder sample ( Supplementary Fig. 6 ). The irradiance spectrum of the total diffuse emission was recorded and its upconversion part was integrated and divided by the excitation light power. The resultant power efficiency of the upconversion by thermal radiation reaches 16% at an excitation power density of 800 W cm −2 ( Fig. 3d ). Since the normalized upconversion quantum yield has often been used in comparing the performances of upconversion materials, we calculated the normalized quantum yields and plotted them as a function of the excitation power density ( Supplementary Fig. 7 ). Our normalized upconversion quantum yields are seen to increase monotonically with increasing excitation power densities. They are not very high in comparison with those reported in other representative works ( Supplementary Table 1 ). Wien’s displacement law [29] states the inverse relationship between a blackbody’s temperature and its radiation peak wavelength. For a blackbody pumped solely by 976-nm light, Wien’s displacement law implies that the higher the blackbody temperature the larger is the portion of the upconversion emission. The portion of the upconversion emission within the total Planckian radiation is plotted as a function of the blackbody temperature in Supplementary Fig. 8 , which clearly depicts the trend inferred from the Wien’s displacement law. This result further suggests that the samples working at higher temperatures can potentially deliver higher power upconversion efficiencies. The powder sample dissipates energy not only through thermal radiation but also through thermal conduction. Thermal convection can be excluded experimentally, for example, by placing the sample in a vacuum chamber. Therefore, the portion of the upconversion emission within the total Planckian radiation determines the theoretical maximum of the upconversion efficiency, and vindicates itself only when thermal conduction is eliminated. In our study, the powder sample irradiated at a maximal blackbody temperature of 2,850 K, which corresponds to a maximal upconversion efficiency of 22% ( Fig. 3d ). The difference in comparison with the measured efficiency of 16% is attributed to thermal conduction loss and can be retrieved by selecting materials with lower thermal conductivities and engineering their architecture to reduce contact thermal conduction. It is straightforward that an oxide at 2,850 K should display thermal expansion in comparison with its volume at room temperature. We indeed observed this thermal expansion in situ both on an optical microscope ( Supplementary Movie 5 ) and on an X-ray diffractometer ( Supplementary Fig. 9 ). The powder sample expands and shrinks when the infrared excitation light is turned on and off, respectively. This observation further confirms the high temperature of the sample under the infrared laser excitation and the thermal radiation nature of the emission. The high rates of the expansion and shrinking processes arise from the fast heating of the particles within the excitation laser beam. We ascertained the stability of the upconversion by thermal radiation at 2,850 K in ambient air by keeping the sample constantly under excitation for 180 min and measuring the upconversion emission intensity every 5 min ( Fig. 3e ). The upconversion emission intensity remained stable without decay. The intensity fluctuates within ±3%, which we believe comes mainly from the instability of the diode laser output. The optical power of the laser was found over a time period of 180 min to have a fluctuation of ±0.63%, and the upconversion emission intensity was measured to be dependent on the excitation optical power nonlinearly, with a power of 3.4 ( Supplementary Fig. 10 ). The nonlinear dependence causes a fluctuation of ±2.1% on the upconversion emission intensity owing to the fluctuation of ±0.63% on the excitation optical power. Stable incandescence from oxides in ambient environment was demonstrated >100 years ago on the Nernst lamp [30] , which used yttria-stabilized zirconia as the incandescent material. The difference lies in that infrared photons are harnessed for heating the oxide in our study, rather than the electric current employed in the Nernst lamp. For the samples calcined at temperatures below 1,400 °C, we observed noticeable emission fluctuation in the earliest 1–2 s of excitation. We speculate that the growth of the crystalline grains within the individual particles during the sample temperature increase in the beginning of the laser excitation gives this emission fluctuation. To validate this hypothesis, X-ray powder diffraction patterns were recorded for the samples with calcination temperatures ranging from 600 to 1,600 °C ( Supplementary Fig. 11 ). The grain sizes were estimated using Scherrer equation [31] , [32] . The result shows a clear trend of larger grain sizes from higher calcination temperatures. The fluctuation at the very beginning of excitation does not affect the steady-state upconversion emission intensity, for which all samples show similar values ( Supplementary Fig. 11 ), despite their different calcination temperatures. This is understandable from the perspective that the high temperature resulting from light absorption eliminates the difference in grain sizes from different calcination temperatures. Effects of the host and sensitizer The irradiance spectra recorded as a function of the excitation power density and their fittings to Planck’s law ( Fig. 3b ) suggest that the sample blackbody temperature saturates at 2,850 K for the excitation power density >760 W cm −2 ( Fig. 3c ). We reason that the sample melting point limits its blackbody temperature. This hypothesis is validated by the melting temperature (2,900 K) of 28 mol% Yb 3+ -doped ZrO 2 reported previously [33] . On the basis of this analysis, together with the consideration of thermal conduction loss above, we postulate that samples with higher melting points and lower thermal conductivities can work at higher blackbody temperatures and dissipate less heat through thermal conduction. They therefore can potentially hit higher upconversion efficiencies. This hypothesis was verified by comparing ZrO 2 with SiO 2 , TiO 2 and Al 2 O 3 as the hosts, from which five orders of magnitude differences were obtained for the upconversion emission intensities ( Fig. 4a ), despite the same sensitizer concentrations and similar absorbance values at the excitation wavelength ( Supplementary Figs 12 and 13 ). Indeed, ZrO 2 possesses the highest melting temperature [33] and a relatively low thermal conductivity [34] among the four types of hosts above ( Fig. 4b ). It sustains the most intense upconversion emission. The lower melting point of SiO 2 and higher thermal conductivities of TiO 2 and Al 2 O 3 explain their lower performance ( Fig. 4b ). We also found the maximal phonon or vibrational energies of the oxide hosts ( Supplementary Tables 2 and 3 ) from previous studies and plotted the power upconversion efficiency as a function of the maximal phonon or vibrational energy to find out their relationship ( Supplementary Fig. 14 ). The power efficiency is seen to decrease as the maximal phonon or vibrational energy is increased, except for SiO 2 , which is probably due to its amorphous nature. 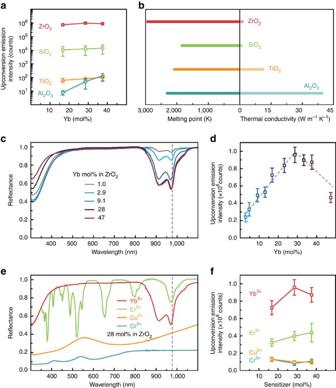Figure 4: Factors affecting the upconversion performance. (a) Upconversion emission intensities from ZrO2, SiO2, TiO2and Al2O3, each doped with 17, 28 and 38 mol% of Yb3+, under 976-nm excitation (1.6 W, 760 W cm−2). ZrO2host delivers two orders of magnitude higher upconversion intensities than SiO2and four to five orders of magnitude higher intensities than TiO2and Al2O3. (b) Melting points and thermal conductivities of the four types of oxide hosts. Oxide hosts with both higher melting points and lower thermal conductivities give higher upconversion emission intensities. (c) Diffuse reflectance spectra of ZrO2doped with Yb3+at increasing concentrations. Changing Yb3+concentration in ZrO2from 1 to 30 mol% increases the absorbance at 976 nm to 0.3. Further increase of Yb3+concentration does not increase the absorbance at 976 nm. (d) Dependence of the upconversion emission intensity on Yb3+concentration in ZrO2. A maximal upconversion emission intensity is observed from 28 mol% Yb3+-doped ZrO2. Samples with higher or lower Yb3+concentrations show lower performance. (e) Diffuse reflectance spectra of ZrO2doped with 28 mol% of Yb3+, Er3+, Cu2+and Cr3+, respectively. (f) Upconversion emission intensities from ZrO2doped with Yb3+, Er3+, Cu2+and Cr3+, with the concentrations of each sensitizer being 17, 28 and 38 mol%, under 976-nm excitation (1.6 W, 760 W cm−2). The upconversion emission intensities do not follow the trend of the light absorbance values at 976 nm, implying the effect of the different sensitizers on the melting point and thermal conductivity of the host. The full height of the vertical error bars corresponds to one s.d. of the measured upconversion emission intensities. Figure 4: Factors affecting the upconversion performance. ( a ) Upconversion emission intensities from ZrO 2 , SiO 2 , TiO 2 and Al 2 O 3 , each doped with 17, 28 and 38 mol% of Yb 3+ , under 976-nm excitation (1.6 W, 760 W cm −2 ). ZrO 2 host delivers two orders of magnitude higher upconversion intensities than SiO 2 and four to five orders of magnitude higher intensities than TiO 2 and Al 2 O 3 . ( b ) Melting points and thermal conductivities of the four types of oxide hosts. Oxide hosts with both higher melting points and lower thermal conductivities give higher upconversion emission intensities. ( c ) Diffuse reflectance spectra of ZrO 2 doped with Yb 3+ at increasing concentrations. Changing Yb 3+ concentration in ZrO 2 from 1 to 30 mol% increases the absorbance at 976 nm to 0.3. Further increase of Yb 3+ concentration does not increase the absorbance at 976 nm. ( d ) Dependence of the upconversion emission intensity on Yb 3+ concentration in ZrO 2 . A maximal upconversion emission intensity is observed from 28 mol% Yb 3+ -doped ZrO 2 . Samples with higher or lower Yb 3+ concentrations show lower performance. ( e ) Diffuse reflectance spectra of ZrO 2 doped with 28 mol% of Yb 3+ , Er 3+ , Cu 2+ and Cr 3+ , respectively. ( f ) Upconversion emission intensities from ZrO 2 doped with Yb 3+ , Er 3+ , Cu 2+ and Cr 3+ , with the concentrations of each sensitizer being 17, 28 and 38 mol%, under 976-nm excitation (1.6 W, 760 W cm −2 ). The upconversion emission intensities do not follow the trend of the light absorbance values at 976 nm, implying the effect of the different sensitizers on the melting point and thermal conductivity of the host. The full height of the vertical error bars corresponds to one s.d. of the measured upconversion emission intensities. Full size image As expected, the sensitizer affects the upconversion through its absorption capability to the excitation light. Increasing Yb 3+ concentration in ZrO 2 from 0 to 30 mol% raises the sample absorbance at 976 nm ( Fig. 4c and Supplementary Fig. 15 ), until the absorbance saturates at 0.3 (50% of incident light being absorbed). Further increasing sensitizer concentration does not increase the absorbance. This result might arise from the diffuse reflection on the powder surface induced by the large refractive index difference between air and the oxide, although its full understanding has remained elusive to us. Architectures facilitating light coupling into the oxide host can potentially improve the upconversion performance by increasing light absorption. Echoing with the absorbance, the upconversion emission intensity ( Fig. 4d ) also increases as Yb 3+ concentration is increased from 0 to 30 mol%. Intriguingly, the upconversion intensity decreases when Yb 3+ concentration is further increased. Previous studies suggest that increasing Yb 3+ concentration above 30 mol % lowers the melting temperature [33] of the sample. Referring to the correlation of poor upconversion with low melting points explains the decrease in the upconversion intensity when Yb 3+ concentration is increased above 30 mol%. The sensitizer is not limited to Yb 3+ . Other sensitizers that can absorb infrared light also work. We exemplified this point using Er 3+ , Cu 2+ and Cr 3+ , other than Yb 3+ , as the sensitizers for 976-nm light ( Fig. 4e,f ) and using Nd 3+ , Dy 3+ , Er 3+ and Tm 3+ as the sensitizers for 808-nm light ( Supplementary Fig. 16 ). Sensitizers that are responsive in different spectral regions can potentially be combined together to achieve broadband absorption of infrared solar radiation. Among these sensitizers, transition metal ions Cr 3+ and Cu 2+ are noteworthy. They are not only cheaper than lanthanides, but also exhibit broadband absorption themselves. What calls for special attention is that doping a sensitizer inevitably alters the thermal conductivity, melting point and refractive index of a host, especially at high doping levels (>10 mol%), therefore affecting the upconversion performance as a whole. Examples can be found in ZrO 2 sensitized with 28 mol% of Nd 3+ , Dy 3+ , Er 3+ and Tm 3+ , among which the upconversion emission intensities are correlated monotonically to the atomic numbers of the sensitizers, rather than their absorbance at the excitation wavelength ( Supplementary Fig. 16 ). We reason that the diminishing ionic radii following the lanthanide contraction lead to strengthened metal–oxygen bonds, and therefore to higher melting temperatures. Further, balancing between the light absorption and thermal properties remains a fruitful task, which echoes with abundant studies on high-temperature thermally isolating materials. Being curious about the performance of the upconversion by thermal radiation in comparison with the state-of-the-art NaYF 4 co-doped with lanthanide ions, we synthesized a bulk sample of hexagonal-phase NaYF 4 :Yb 3+ ,Er 3+ following recent reports [15] , [35] and measured the upconversion intensity as a function of the excitation power density at 976 nm. The results are plotted together with those from Yb 3+ -doped ZrO 2 in Supplementary Fig. 17 . Thermal radiation offers higher upconversion intensities at excitation power densities between 200 and 800 W cm −2 . At lower excitation power densities, the NaYF 4 :Yb 3+ ,Er 3+ sample performs better. Therefore, we reckon the upconversion by thermal radiation to be more preferable for concentrated solar radiation [36] , [37] . The different power dependence behaviours between our sample and the NaYF 4 :Yb 3+ ,Er 3+ sample are attributed to their distinct upconversion mechanisms. Upconversion through thermal radiation requires the blackbody temperature to be above ~1,500 K, so that the upconversion part becomes significant within the entire Planckian radiation ( Supplementary Fig. 8 ). This in turn requires high excitation power densities. In comparison, for energy transfer upconversion materials, such as NaYF 4 :Yb 3+ ,Er 3+ , upconversion arises from the photoluminescence of activator ions, which are excited through the energy transfer from sensitizer ions. The minimal excitation power densities required for enabling the energy transfer from sensitizer ions to activator ions and for observing the upconversion emission is relatively low. In addition, for the NaYF 4 sample, the excited states of Er 3+ ions can be completely filled at high excitation power densities, which prevents Er 3+ ions from further accepting energy from Yb 3+ ions. This is known as the saturation effect [38] , which promotes nonradiative decay. As a result, the NaYF 4 sample performs better than our sample at low excitation power densities, while at high excitation power densities, our sample is superior. All of our upconversion measurements described above were performed under the excitation of coherent, narrowband laser light sources. An essential aspect in the development of new upconversion approaches and materials for harvesting low-energy solar photons is their ability to work directly under sunlight and upconvert low-energy photons to high-energy ones [2] , [6] , [7] , [13] , [14] , [18] , [19] , [20] , [39] . We therefore further demonstrated the feasibility of our thermal radiation-based approach towards sunlight. Since the optical power density of sunlight is about four orders of magnitude smaller than that of the laser light used in our above measurements, the sunlight was concentrated with a biconvex lens at a concentration factor of 8,600. A 715-nm long-pass filter was utilized to block ultraviolet and visible sunlight and allow for infrared sunlight to pass with high transmittance. We examined the ZrO 2 samples doped with lanthanide ions, Yb 3+ , Er 3+ , Tm 3+ , Dy 3+ and Nd 3+ , and transition metal ions, Cr 3+ and Cu 2+ , at 28 mol%. The samples doped with the lanthanide ions have narrowband light absorption, while those doped with the transition metal ions exhibit broadband absorption ( Supplementary Fig. 18a ). Under the concentrated and filtered sunlight excitation, only the Cr 3+ - and Cu 2+ -doped ZrO 2 samples were seen to glow ( Fig. 5a–c ). To better ascertain the reason for the difference in the glowing behaviours, we integrated the solar irradiance that was absorbed by the doped samples over the spectral range from 715 to 2200, nm according to the diffuse reflectance spectra and the solar irradiance spectrum ( Supplementary Fig. 18 ). The solar power densities absorbed by the samples doped with the transition metal ions were found to be 5–10 times higher than those doped with the lanthanide ions. The glowing behaviour under infrared sunlight excitation is comparable to that under the 976-nm laser excitation ( Supplementary Fig. 19 ). The glowing spots under infrared sunlight excitation appear weaker than those under the laser excitation, which is consistent with the fact that the determined blackbody temperatures in the former are lower than those in the latter by 800–1,000 K. This is reasonable because the optical power density of the concentrated and filtered sunlight is still smaller than that of the laser. The glowing observed under infrared sunlight clearly shows the feasibility of our thermal radiation-based route to the absorption and upconversion of low-energy solar photons into high-energy ones. In addition, the concentration factor of our biconvex lens is 8,600. If we consider that solar concentrators with concentration factors as high as 84,000 have been reported [36] , [37] , our ZrO 2 samples doped with narrowband lanthanide ions and broadband transition metal ions are also expected to glow under the filtered sunlight that is concentrated at higher factors. 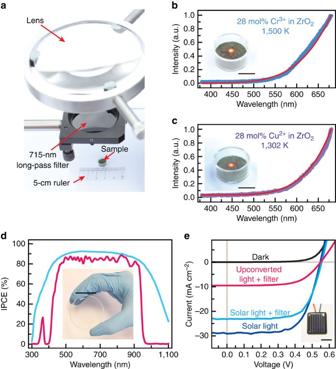Figure 5: Upconversion-glowing under sunlight excitation and upconversion solar cell performance. (a) Photograph of the measurement setup under sunlight excitation. The lens has a diameter of 10.2 cm and a focal length of 18 cm. The sunlight at the measurement time and location had an optical power density of 0.09 W cm−2. It was focused onto the sample surface at a spot size of 1.1±0.1 mm in diameter, with 51% of the optical power being filtered off. The resultant optical power densities absorbed by the samples were 289 W cm−2for Cr3+-doped ZrO2and 205 W cm−2for Cu2+-doped ZrO2. (b) Upconversion emission spectrum (blue) and glowing photograph (inset; scale bar, 0.5 cm) of 28 mol% Cr3+-doped ZrO2under sunlight excitation. The fitting (red) according to the Planck’s law gave a blackbody temperature of 1460±110 K. (c) Upconversion emission spectrum (purple) and glowing photograph (inset; scale bar, 0.5 cm) of 28 mol% Cu2+-doped ZrO2under sunlight excitation. The blackbody temperature obtained from the fitting (red) is 1,300±60 K. (d) Incident photon-to-current conversion efficiency spectra of a commercial polycrystalline Si solar cell under simulated AM1.5 solar light (cyan) and with a 950-nm short-pass filter (pink). The inset is the photograph of the short-pass filter (scale bar, 3 cm). The transmittance of the filter at 976 nm is 0.2%. (e) Current density–voltage curves of the Si solar cell under AM1.5 solar light (blue) with the short-pass filter (cyan), under the upconverted white light with the short-pass filter (pink) and in dark (black). The upconverted white light came from 28 mol% Yb3+-doped ZrO2under the 976-nm laser excitation (1.6 W, 760 W cm−2). The inset is the photograph of the polycrystalline Si solar cell (scale bar, 1 cm). Figure 5: Upconversion-glowing under sunlight excitation and upconversion solar cell performance. ( a ) Photograph of the measurement setup under sunlight excitation. The lens has a diameter of 10.2 cm and a focal length of 18 cm. The sunlight at the measurement time and location had an optical power density of 0.09 W cm −2 . It was focused onto the sample surface at a spot size of 1.1±0.1 mm in diameter, with 51% of the optical power being filtered off. The resultant optical power densities absorbed by the samples were 289 W cm −2 for Cr 3+ -doped ZrO 2 and 205 W cm −2 for Cu 2+ -doped ZrO 2 . ( b ) Upconversion emission spectrum (blue) and glowing photograph (inset; scale bar, 0.5 cm) of 28 mol% Cr 3+ -doped ZrO 2 under sunlight excitation. The fitting (red) according to the Planck’s law gave a blackbody temperature of 1460±110 K. ( c ) Upconversion emission spectrum (purple) and glowing photograph (inset; scale bar, 0.5 cm) of 28 mol% Cu 2+ -doped ZrO 2 under sunlight excitation. The blackbody temperature obtained from the fitting (red) is 1,300±60 K. ( d ) Incident photon-to-current conversion efficiency spectra of a commercial polycrystalline Si solar cell under simulated AM1.5 solar light (cyan) and with a 950-nm short-pass filter (pink). The inset is the photograph of the short-pass filter (scale bar, 3 cm). The transmittance of the filter at 976 nm is 0.2%. ( e ) Current density–voltage curves of the Si solar cell under AM1.5 solar light (blue) with the short-pass filter (cyan), under the upconverted white light with the short-pass filter (pink) and in dark (black). The upconverted white light came from 28 mol% Yb 3+ -doped ZrO 2 under the 976-nm laser excitation (1.6 W, 760 W cm −2 ). The inset is the photograph of the polycrystalline Si solar cell (scale bar, 1 cm). Full size image One underlying motivation in developing upconversion materials with high upconversion efficiencies is to enhance the usage of infrared solar photons. In this regard, we finally examined whether the higher-energy photons upconverted by our material from infrared photons can be absorbed by commercial Si solar cells to generate electrical power. Owing to the limitations in concentrating natural sunlight, as well as, the simulated solar light, we chose to use the 976-nm laser to excite our upconversion material, 28 mol% Yb 3+ -doped ZrO 2 , for this experiment. The measurement setup was composed of a parabolic reflection cup, a 950-nm short-pass filter, and a Si solar cell ( Supplementary Fig. 20 ). The incident photon-to-current conversion efficiency of the used Si solar cell is ~90% in the spectral range from ~450 to 900 nm ( Fig. 5d ). The power conversion efficiency of the cell is 12%. The 950-nm short-pass filter has high light transmittances from ~475 to 900 nm, as shown by the slight reduction in the incident photon-to-current conversion efficiency values in this spectral range after the insertion of the filter. Under the excitation of the 976-nm laser at 1.60 W, the power conversion efficiency of the entire system relative to the excitation power of the 976-nm laser was found to be 0.63% ( Supplementary Table 4 ). We also calculated the external quantum efficiency and the normalized external quantum efficiency of our system, since both are often utilized in characterizing the upconversion photovoltaic performances of different materials. The former is defined as the ratio between the number of collected charge carriers by the solar cell and the number of photons incident on the upconverter, and the latter is the external quantum efficiency divided by the excitation light power density. Compared with the values reported in recent representative studies, our external quantum efficiency, 2.0%, is relatively high, but our normalized external quantum efficiency, 2.6 × 10 −5 , is relatively low ( Supplementary Table 5 ). Our low normalized external quantum efficiency is mainly caused by the high excitation power density used for upconversion. To visually demonstrate the upconversion photovoltaic performance of our material, we used the electricity that was generated by Si solar cells to drive a green light-emitting diode ( Supplementary Fig. 21 ) and a miniature motor with a small propeller ( Supplementary Movie 6 ). The Si solar cells were irradiated by the upconverted light from 28 mol% Yb 3+ -doped ZrO 2 , which was excited by the 976-nm laser at 1.60 W. The diode and the motor could be switched on and off repeatedly by turning on and off the 976-nm laser. Possible geometrical configurations for applying our upconversion material to photovoltaic applications are proposed schematically in Supplementary Fig. 22 . In these proposed configurations, bifacial solar cells are utilized. Low-energy photons that pass through the solar cell without being absorbed are focused with a lens, a parabolic concentrator or a micro-lens array onto the upconversion material. The upconverted high-energy photons are then directed back to the solar cell. Sample synthesis All doped oxides were prepared using a sol–gel method, with organometallic compounds as the oxide precursors and high-purity metal chlorides as the sensitizer precursors. More preparation details are provided in Supplementary Methods . Optical characterization Two continuous wave semiconductor diode lasers, with working wavelengths of 976 and 808 nm, respectively, were utilized as the excitation sources. The laser spot size was determined by shining the collimated laser light onto a diffuse reflection surface, fitting the captured spot image with a two-dimensional Gaussian peak, and finding the lateral sizes corresponding to 1/ e of the peak value along the two directions ( Supplementary Fig. 23 and Table 6 ). Emission spectra were acquired on a monochromator that was coupled to a Si charge-coupled device camera working in the range from 350 to 850 nm and an InGaAs camera working in the range from 1,050 to 1,600 nm. Emission spectra (photon flux as a function of wavelength) were multiplied by photon energies to obtain the corresponding irradiance spectra (light power as a function of wavelength). An optical setup was custom-built for comparing the upconversion emission intensities of different samples. For each sample, 30 measurements were performed on different spots. The emission intensity from each spot was calculated by integrating the emission spectrum from 380 to 900 nm. The emission intensity of the sample was obtained by averaging the 30 intensity values. The power upconversion efficiency is defined as the power of the upconversion emission divided by the power of the absorbed excitation light. The total power of the upconversion emission under 976-nm excitation was collected using a 75-mm-diameter integrating sphere coupled to a spectrophotometer working in the range from 380 to 970 nm. The power of the absorbed excitation light was calculated from the excitation light power times the absorption fraction (1−diffuse reflectance) at 976 nm. The spot size under the concentrated sunlight was determined by placing a flat black silicone rubber plate at the focus point of the biconvex lens for ~1 s, recording the optical image of the burned spot, and then measuring the diameter of the spot on the optical image ( Supplementary Fig. 24 ). The setup for examining the upconversion photovoltaic performance was composed of a Si solar cell, a 950-nm short-pass filter, a parabolic reflection cup and the 976-nm laser. The upconversion powder material was placed at the bottom of the cup, which was covered with the filter. The solar cell was positioned right above the filter. A small hole was opened on the side wall of the cup for introducing the excitation laser light. The electricity generated from the solar cells under the upconverted light was also used to drive a green light-emitting diode and a miniature motor with a small propeller. More optical characterization details are provided in Supplementary Methods . Fitting the irradiance spectra with Planck’s law The measured irradiance spectra were fitted according to Planck’s law on the basis of the function below to determine the sample temperature: where T is the absolute temperature of the blackbody, λ is wavelength, a is a fitting parameter, h is the Planck constant, c is the speed of light and k B is the Boltzmann constant. How to cite this article : Wang, J. et al . Photon energy upconversion through thermal radiation with the power efficiency reaching 16%. Nat. Commun. 5:5669 doi: 10.1038/ncomms6669 (2014).